Patterns and flow in frictional fluid dynamics Pattern-forming processes in simple fluids and suspensions have been studied extensively, and the basic displacement structures, similar to viscous fingers and fractals in capillary dominated flows, have been identified. However, the fundamental displacement morphologies in frictional fluids and granular mixtures have not been mapped out. Here we consider Coulomb friction and compressibility in the fluid dynamics, and discover surprising responses including highly intermittent flow and a transition to quasi-continuodynamics. Moreover, by varying the injection rate over several orders of magnitude, we characterize new dynamic modes ranging from stick-slip bubbles at low rate to destabilized viscous fingers at high rate. We classify the fluid dynamics into frictional and viscous regimes, and present a unified description of emerging morphologies in granular mixtures in the form of extended phase diagrams. In their landmark paper from 1958, Saffman and Taylor introduced the Hele-Shaw cell, two parallel plates separated by a small gap, as an idealized model system for the study of hydrodynamic interfacial instabilities [1] , [2] . This simple setup has since provided important insights into fundamental aspects of branching patterns [3] , [4] , [5] , [6] , [7] , [8] , and into the flow behaviour of non-Newtonian fluids typically found in consumer products and industrial materials [9] , [10] , [11] , [12] . Recently, several authors have considered displacement patterning in granular suspensions, in which care is taken to match the density of the grains and the host fluid [13] , [14] , [15] . Displacement dynamics in settling granular mixtures, in which inter-particle friction has a central role, have received less attention. Such 'frictional fluids' are ubiquitous in nature and engineering. For example, they have a key role in landslides, where fluidization causes the rheology to jump rapidly from solid- to fluid-like behaviour. Of interest in engineering applications is the role of frictional granular mixtures in oil and gas recovery, and potentially for processes linked to CO 2 geo-sequestration. From a materials science point of view, frictional fluids are strongly related to such complex materials as Bingham or yield stress fluids, in which non-Newtonian behaviour reflects jamming mechanisms on the molecular level that resemble static friction on the macro-level. In Liu and Nagel's generalized description of jamming, an arrested assembly of grains can be fluidized through dilation or by increasing the applied stress [16] , [17] , [18] . The origin of jamming is closely linked to the presence of force chains within the packing [19] , [20] , and the unjamming, or yielding, occurs as grain–grain contacts become mobilized, leading to destabilization and buckling of the load carrying force chains [21] . Recently Fall et al . found that many puzzling phenomena observed for dense granular suspensions, such as shear banding and a yield stress well below the close packing limit, can be attributed to sedimentation or creaming induced by gravity [22] . Only the slightest density mismatch between the grains and the fluid has a profound impact on the rheology as close-packed regions form where normal forces create force chains that stabilize the system. The majority of dense noncolloidal mixtures will thus display frictional responses induced by gravity, especially at low flow velocities where hydrodynamic interactions are less dominant [23] . Here we use a generic granular material that settles in a Newtonian fluid to explore the displacement dynamics of a system with both rheological and tribological characteristics. We map the dynamic response of the frictional fluid as it is displaced by air, and we focus on the effects of the granular filling fraction ϕ , system stiffness K and the injection rate q . Several new dynamic modes are uncovered and presented in phase diagrams illustrating the various morphologies and the transitions between them. At low rate, the frictional contacts between grains introduce a kind of intermittent behaviour familiar from processes such as stick-slip sliding [24] , [25] , earthquakes [26] and granular avalanches [27] , [28] , [29] . A transition to the viscous regime is observed as hydrodynamic interactions dominate at high injection rate. Finally, we consider displacement dynamics as ϕ approaches 1, where the system takes on the properties of a more or less solid porous medium. Frictional flow at low rate Pressurized air is injected into a confined, settled granular mixture using a syringe pump driven at a constant rate ( Fig. 1a ). The height of granular material in the gap depends on the initial filling fraction ϕ of the mixture (where ϕ is normalized with the filling fraction of close-packed grains). The syringe contains a reservoir of air of volume V air . 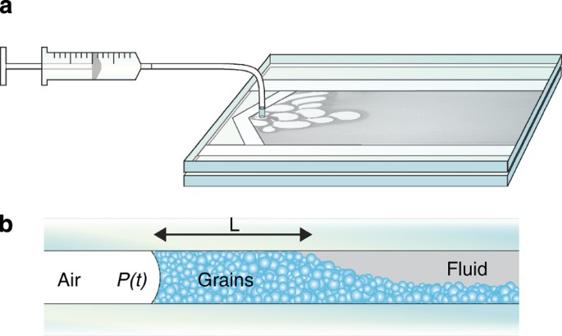Figure 1: Setup and displacement process. (a) Air is slowly injected into a linear Hele-Shaw cell loaded with polydisperse glass beads (∼100 μm diameter) submersed in a water/glycerol solution. The gap is Δz=0.5 mm and the cell forms a channel 20 cm wide and 30 cm long. The granular material settles after loading. (b) The invading air/fluid interface accumulates a front of close-packed grains in the gap between the plates. The air/fluid interface advances and accumulates a front of compacted granular material of thickness L as illustrated in Figure 1b . Here, horizontal stress imposed by capillary forces at the interface is transmitted through force chains within the packing. As the granular packing is unable to dilate, the normal force on the confining plates increases. We adopt a Janssen model [30] for the stress in the packing, such that σ zz = κσ xx , where κ is the Janssen proportionality constant giving the ratio of transverse to in-plane granular pressure. The frictional stress σ at the interface that must be overcome to move the front is derived [31] , and takes the form σ ∼ Δ z [exp( L /Δ z )−1]. Figure 1: Setup and displacement process. ( a ) Air is slowly injected into a linear Hele-Shaw cell loaded with polydisperse glass beads ( ∼ 100 μm diameter) submersed in a water/glycerol solution. The gap is Δ z =0.5 mm and the cell forms a channel 20 cm wide and 30 cm long. The granular material settles after loading. ( b ) The invading air/fluid interface accumulates a front of close-packed grains in the gap between the plates. 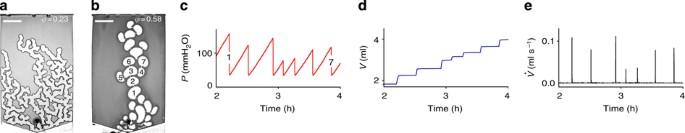Figure 2: Friction fingers and stick-slip bubbles. (a) At low granular filling fractionϕ, air slowly displaces the granular-fluid mixture in a creeping fingering process. (b) A transition to highly intermittent dynamics occurs at highϕ. A single bubble of air suddenly inflates after a long static period. Both experiments:Vair=30 ml,q=0.02 ml min−1, scale bar, 5 cm. (c) Gas pressure, (d) invaded volumeVand (e) the flow rateas a function of time for the bubbles labelled 1–7 inb(Supplementary Movie 1). Full size image At low granular filling fraction the injected air advances in a slow and quasi-continuous fingering process where side-branching of fingers and a random growth direction produces a branched labyrinthine structure as seen in Figure 2a . The front of compacted grains, compiled by the advancing interface, can be seen along the entire front as a narrow, dark band. We have previously shown that a characteristic finger width emerges as a result of the force balance between the gas pressure on the inside of the finger and the capillary forces and friction at the interface. This characteristic width gives rise to the uniform wavelength of the labyrinths seen in fully drained systems [32] and decreases with increasing ϕ . Figure 2: Friction fingers and stick-slip bubbles. ( a ) At low granular filling fraction ϕ , air slowly displaces the granular-fluid mixture in a creeping fingering process. ( b ) A transition to highly intermittent dynamics occurs at high ϕ . A single bubble of air suddenly inflates after a long static period. Both experiments: V air =30 ml, q =0.02 ml min −1 , scale bar, 5 cm. ( c ) Gas pressure, ( d ) invaded volume V and ( e ) the flow rate as a function of time for the bubbles labelled 1–7 in b ( Supplementary Movie 1 ). Full size image The low rate means that viscous forces are negligible. Capillary and friction forces act locally and thereby effectively screen the fingers from their surroundings. The characteristic finger scale is therefore independent of channel width, contrary to what is generally observed in viscous fingering in most Newtonian and non-Newtonian fluids [3] , [10] , [33] . One exception is viscous fingering in yield stress fluids, in which the finger width at low rate is found to be independent of channel width and velocity, and instead influenced by surface tension and the yield stress of the material [12] . This similarity in behaviour is perhaps not surprising as both yield stress and frictional fluids are governed by threshold-limited dynamics associated with the yield stress and the static friction, respectively. When we increase ϕ above a threshold value, the dynamics changes dramatically and a different morphology emerges ( Fig. 2b ). The advancement of the interface is no longer slow and creeping, instead its motion becomes highly intermittent. The front remains stationary for an extended period, followed by a sudden displacement of the granular-fluid mixture by a burst of air in the shape of a bubble. The displacement progresses bubble by bubble in a stick-slip manner. During the static periods, the gas pressure increases linearly as the air is compressed by the constant, slow driving of the piston ( Fig. 2c ). The gas pressure is balanced by the frictional stress from the jammed granular front. As the pressure builds, the weakest point along the front finally yields, and the pressurized air invades rapidly through a narrow neck before expanding radially. The air decompresses and the expansion slows and stops. The granular material accumulated by the interface settles and gradually compacts into a jammed front where once again the weakest point determines the location and yield pressure for the next bubble (and therefore its size). Figure 2d,e shows the volume invaded by the bubbles and the flow rate, respectively. In the spring-block sliding friction problem, the elasticity of the spring enables stick-slip motion. Baumberger et al . found a bifurcation from stick-slip to continuous sliding by increasing the stiffness of the spring [24] . In our system, the elasticity is provided by the compression of the reservoir volume of air being injected, V air . We use Boyle's law for isothermal expansion of an ideal gas to find the pressure drop Δ P associated with the expansion of a bubble of volume Δ V , where P 0 is the background pressure. We define the volumetric stiffness of the system as K = P 0 / V air . There is an additional small contribution (≈240 Pa) from the out-of-plane capillary pressure, which accounts for the relaxation pressure after each bubble creation (see Fig. 2c ). This pressure contribution is constant and is included in P 0 . 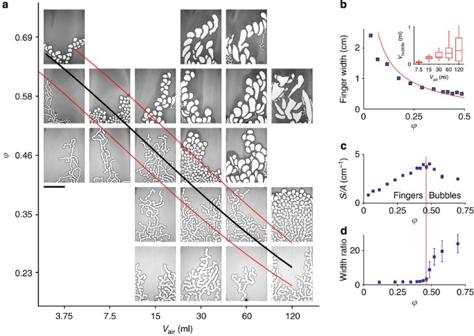Figure 3: Frictional dynamics transition. (a) Displacement structures obtained by varyingϕandVair, keepingqconstant (0.03 ml min−1). Frictional fingers are stable at low filling fraction and elasticity, whereas stick-slip bubbles prevail at highϕandVair. The theoretical model for the phase boundary is superimposed on the images (black line), including the effect of a ±10% variation in the friction coefficientμ(red lines). Scale bar, 10 cm. (b) The finger width decreases with increasingϕ(squares, experiments; solid line, theory). Inset: Bubble size increases withVair, but varies considerably as evident from this box plot showing median, quartiles and extremes (whiskers).ϕ=0.58 for this data set. (c) Interface to area ratioS/A. Error bars on two data points denote standard deviations in replicate experiments. (d) Ratio of adjacent maximum to minimum width plotted as a function ofϕ. Mean and standard deviation obtained by 20 random measurements. Red line: theoretical result for the phase boundary. Figure 3a shows images from experiments probing a phase space of ϕ and V air . The fingering dynamics is stable for low filling fraction and small air volumes (high stiffness). A transition to the highly intermittent bubble phase can be achieved by increasing ϕ or by making the system more elastic (increasing V air ). This result mirrors the behaviour of the sliding block, in which the bifurcation from stick slip to smooth sliding occurs above a critical stiffness/weight ratio [34] . Figure 3: Frictional dynamics transition. ( a ) Displacement structures obtained by varying ϕ and V air , keeping q constant (0.03 ml min −1 ). Frictional fingers are stable at low filling fraction and elasticity, whereas stick-slip bubbles prevail at high ϕ and V air . The theoretical model for the phase boundary is superimposed on the images (black line), including the effect of a ±10% variation in the friction coefficient μ (red lines). Scale bar, 10 cm. ( b ) The finger width decreases with increasing ϕ (squares, experiments; solid line, theory). Inset: Bubble size increases with V air , but varies considerably as evident from this box plot showing median, quartiles and extremes (whiskers). ϕ =0.58 for this data set. ( c ) Interface to area ratio S / A . Error bars on two data points denote standard deviations in replicate experiments. ( d ) Ratio of adjacent maximum to minimum width plotted as a function of ϕ . Mean and standard deviation obtained by 20 random measurements. Red line: theoretical result for the phase boundary. Full size image The finger tip curvature R c is a result of the competing influences of the effective surface tension and the frictional stress from the granular front [32] , and consequently the characteristic width of the air fingers decreases with ϕ as shown in Figure 3b . Here, the finger width is measured as A /( S /2) where A is the area occupied by the finger and S is the interface length as determined by image analysis. The solid line shows the theoretical result for the finger width 2 R , where we have used μ =0.53 for the effective granular friction coefficient and κ =0.8 to fit the model to the experimental data. The size of the bubbles is seen to grow both with increasing ϕ (higher friction causes higher yield pressures) and increasing V air (larger reservoir of air available for decompression). The inset in Figure 3b shows statistics of bubble volumes measured for a series of experiments with increasing V air . There is considerable variation in bubble size within each experiment, and the width of the size distribution increases along with the median size for increasing ϕ and V air . Note that the finger growth, even though it appears continuous, is in fact a result of incremental movements caused by individual stick-slip events. The transition from fingers to bubbles therefore does not represent a fundamental shift in dynamic state, rather, it is a qualitative change in pattern morphology governed by the magnitude of each slip event. Theoretically, we define the phase boundary as the point where the expanding air volume Δ V increases above , corresponding to a circular bubble of radius equal to the radius of curvature of the finger. Further, we assume that the static friction of the jammed granular layer is fully demobilized during a slip event such that Δ P =− σ ( L ). Having found the characteristic curvature R c , equation (1) gives or, using the expression for σ ( L ) that we find in ref. 31 , where γ is the effective surface tension of the fluid, ρ the mass density of the granular packing corrected for the buoyancy of the fluid and g the acceleration of gravity. The thickness of the granular front depends on the filling fraction and the finger curvature, L = ϕR c /(1− ϕ ). The above prediction for the phase boundary, expressed as the minimum required air volume for bubbles given the filling fraction, is plotted in Figure 3a . The model pinpoints the transition well, especially considering its simplifying assumptions. The phase boundary is sensitive to the effective friction coefficient of the granular material as shown by the red lines corresponding to ±10% variation in μ . Two 'order parameters' are introduced; (1) the interface length divided by the area occupied by the structure, S / A , and (2) the ratio between adjacent maximum/minimum widths, which for fingers correspond to variation in finger width, and for bubbles, their average diameter divided by the width of the narrow neck from which they inflated. Figure 3c shows that the interface length per area grows linearly with ϕ until the transition point and then decreases because of the fact that circular structures minimizes surface. The width ratio, plotted in Figure 3d , is more sensitive to observed differences in morphology at the transition point. Both order parameters demonstrate that the crossover from quasi-continuous fingers to stick-slip bubbles occurs as a continuous transition over a fairly narrow region of the phase space. Transition from frictional to viscous dynamics The rate dependency of the displacement patterning is probed in a series of experiments spanning four decades in the injection rate q ( Fig. 4 ). Several new dynamic modes and morphologies emerge, and we classify these broadly into a frictional regime and a viscous regime. 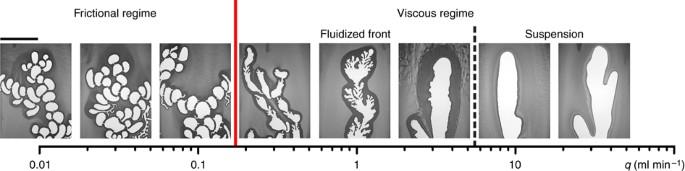Figure 4: Rate dependency. Displacement structures as a function of injection rateq. Frictional stick-slip flow at low rates gives way to continuous motion as viscous forces fluidize the accumulated front, and, at yet higher rates, suspends the granular material (ϕ=0.58,Vair=30 ml, scale bar, 10 cm). (Supplementary Movie 2). Figure 4: Rate dependency. Displacement structures as a function of injection rate q . Frictional stick-slip flow at low rates gives way to continuous motion as viscous forces fluidize the accumulated front, and, at yet higher rates, suspends the granular material ( ϕ =0.58, V air =30 ml, scale bar, 10 cm). ( Supplementary Movie 2 ). Full size image At low-flow rates the interface motion is slow enough that the grains accumulated by the front have time to expel interstitial fluid, settle onto the slowly advancing front, and form frictional contacts. As demonstrated in the previous section, this friction gives rise to intermittent behaviour, manifesting itself in the stick-slip bubble pattern, or alternatively, as frictional fingering in the case of low filling fraction and elasticity (see Fig. 3a ). As the injection rate is increased, viscous forces start to dominate the interactions, bringing the system to the viscous, or continuous dynamics, regime ( Fig. 4 ). The critical injection rate for the transition to continuous motion can be formulated as a requirement that the moving granular front is kept fluidized and prevented from jamming. In other words, the fluid forces inside the dense granular packing must exceed the friction caused by the weight of the grains: | ∇ P |> μρg , where ∇ P now is the fluid pressure gradient. Invoking Darcy's law and the Kozeny–Carman relation we find where k ( ξ ) is the permeability as a function of the porosity ξ and η is the viscosity of the fluid. Equation (4) predicts a lower bound of q c =0.05 ml min −1 for the transition from the frictional to the viscous regime. This value represents the lowest flow rate at which continuous motion is possible, but the system is likely to be unstable since any random stick-slip event would lead to a transient high flow, followed by slow flow allowing friction to re-mobilize. This is consistent with the experimental observations, in which the transition is seen to occur above 0.1 ml min −1 . Note that q c is independent of ϕ and V air , a result that is broadly supported by experimental results, however, some secondary effects of the elasticity is observed. Again, we highlight the similarities in behaviour to other systems displaying intermittency, in which, for example, the sliding block makes a transition from stick-slip to continuous smooth motion as the driving velocity is increased [24] , and similar rate-dependent changes of dynamic state are also observed for granular avalanches in rotating drums [28] . In addition, we find that the transition from frictional (intermittent) to viscous (continuous) dynamics is not abrupt, as there is a significant crossover region exemplified by the experiment at 0.3 ml min −1 in Figure 4 , where the dynamics alternates between continuous motion and occasional jamming. This transitional mode has parallels to the kind of temporal intermittency observed as an intermediate stage in frictional sliding [35] and granular avalanches [28] . We now focus on the viscous regime, in which, at intermediate flow rates, the velocity of the invading interface is high enough to fluidize the accumulated packing and keep it from establishing frictional contacts. Note that the hydrodynamic interactions occur mainly between grains in close proximity, such that a distinct band of compacted granular material forms around the displacement front, whereas the granular layer in the rest of the cell remains undisturbed by the fluid flow in the channel (0.3–3 ml min −1 , Fig. 4 ). The striking 'coral' structures (1 ml min −1 ) grow in a process that alternates between large-scale radial expansion and sprouting of narrow fingers. The one narrow finger that gets ahead of the rest accelerates and grows into a bubble. As the bubble expands radially, the front velocity slows and the packing starts to compactify. This in turn causes the effective viscosity of the fluidized front to increase and the pressure to rise, and soon the interface becomes unstable again and new fingers develop. These fingers are akin to viscous fingers where the less viscous air penetrates the fluidized granular material driven by the pressure gradient over the compacted front. The instability is amplified as the fingers in motion keep the granular material ahead highly fluidized, whereas slower regions compactify further, causing higher local viscosity, deceleration and so on. As we increase the injection rate beyond ∼ 10 ml min −1 , the system undergoes yet another transition, this time to the more familiar pattern formation process of viscous fingering. The transition occurs when the fluid flow in the channel is fast enough that fluid drag overcomes the gravitational sedimentation and re-suspends the granular layer, which has settled on the lower glass plate. The images show that the granular material in the entire cell is set in motion, and there is therefore no formation of a compacted granular front around the invading interface. The granular-fluid mixture now effectively acts like a suspension, and the dynamics is dominated by the viscous response to the flow in the channel and the Saffman-Taylor instability [1] , [14] . We find an early destabilization and branching of the viscous fingers (30 ml min −1 ), which has been observed by other authors, and attributed to noise due to the discrete nature of the granular medium [13] . From frictional fluid to porous medium As we extend the investigation to increasingly high filling fractions, the system changes characteristics from fluid- to solid-like behaviour. We find a transition to fracturing from approximately ϕ >0.9 ( Fig. 5a ), where the poorly compacted granular material can be described as a deformable, or weak, porous medium. Fracturing has previously been observed in viscoelastic fluids [9] and density-matched suspensions of grains [14] . The industrial process of hydraulic fracturing is commonly used in oil reservoir engineering [36] , [37] . Note, however, that this typically involves the injection under high pressure of a fracturing fluid with low compressibility, such that the elastic response originates mainly from the in situ medium. 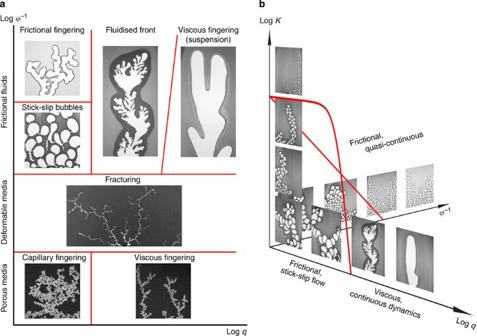Figure 5: Phase space. (a) Tentative phase diagram of morphologies in theϕ−1−qplane extended to theϕ=1 limit corresponding to a close-packed porous medium. Various displacement morphologies in the frictional fluid give way to fracturing atϕ>0.9, followed by a transition to capillary/viscous fingering in porous media (ϕ≈1).The phase boundaries are 'guides to the eye'. The images of capillary and viscous fingering in porous media have been obtained using different experimental setups by other authors38,42. (b) A framework for displacement dynamics in frictional fluids illustrating the transitions between intermittent frictional, quasi-continuous frictional and continuous viscous fluid dynamics. Figure 5: Phase space. ( a ) Tentative phase diagram of morphologies in the ϕ −1 − q plane extended to the ϕ =1 limit corresponding to a close-packed porous medium. Various displacement morphologies in the frictional fluid give way to fracturing at ϕ >0.9, followed by a transition to capillary/viscous fingering in porous media ( ϕ ≈1).The phase boundaries are 'guides to the eye'. The images of capillary and viscous fingering in porous media have been obtained using different experimental setups by other authors [38] , [42] . ( b ) A framework for displacement dynamics in frictional fluids illustrating the transitions between intermittent frictional, quasi-continuous frictional and continuous viscous fluid dynamics. Full size image Ultimately, when the system approaches the close packing limit, the granular material is effectively a rigid porous medium, and the displacement of the fluid progresses pore by pore governed by local capillary and viscous forces [5] , [38] , [39] . At low flow rates, the invasion dynamics is dominated by the threshold capillary pressure fluctuations in the heterogeneous medium, giving rise to a pore scale percolation displacement or capillary fingering ( Fig. 5a , lower left corner). As the flow rate increases, so does the viscous pressure gradient in the channel and the Saffman-Taylor instability gives rise to viscous fingering ( Fig. 5a , lower right corner). The transition between these two regimes can be expressed in terms of the modified capillary number, Ca *, that gives the ratio of the viscous pressure gradient along the channel to the width of the capillary pressure distribution in the porous media [39] , [40] , with the transition at Ca *≈1. The 'frictional fluid' in this study represents a model system for settling granular mixtures where gravity-induced frictional forces have a profound impact on the fluid dynamics. We find that the concept of constitutive behaviour becomes less relevant in the frictional regime, as the dynamics is governed by self-assembled compacted regions with local yield stresses. At low rate, particle–particle contacts form as interstitial fluid between grains is expelled. The frictional response from a compacted front of granular material induces intermittent behaviour, and we find two distinct morphologies, fingers and bubbles, depending on whether the motion occurs incrementally or in large stick-slip events ( Fig. 3a ). Increasing the injection rate results in a series of transitions, first to a continuous displacement mode characterized by a fluidized, or lubricated, front of accumulated material ( Fig. 4 ). Note that stress mediation through the dense granular front now occurs through hydrodynamic interactions rather than solid contacts as in the frictional regime. Therefore, when the injection rate is decreased by a factor of a hundred, and the viscosity increased by the same factor, the same 'coral' pattern results, giving support to the scaling in equation 4 where q c ∼ 1/ η . When the injection rate is increased to the point where the flow in the channel is fast enough to re-suspend the settled material, the well-known Saffman-Taylor instability governs the dynamics, resulting in viscous fingering in the granular suspension [13] , [14] . Figure 5b shows a schematic three dimensional phase diagram illustrating the transitions between frictional bubbles and fingers, and frictional and viscous dynamics in the K – ϕ −1 plane and the K – q plane, respectively. Note that the red lines demarcating the phase boundaries are intended as 'guides to the eye', and that the precise location of the transitions will depend on many factors, including the roughness of the grains, the viscosity of the host fluid and the mass density difference between the grains and the fluid. The phase boundary in the K – ϕ −1 plane is determined theoretically (equation 3), whereas for the K – q plane we find that the transition rate is fairly independent of elasticity up to the point where high stiffness quenches the bubbles, introducing the frictional fingering regime. To elucidate the relationship between the new frictional fluid morphologies that we present here and displacement patterns observed in porous media, we combine our findings with recent results from other authors [14] , [38] , [41] and draw a tentative ϕ −1 – q phase diagram including fracturing, and capillary and viscous fingering in porous media where ϕ ≈1 ( Fig. 5a ). Again, the demarcation lines are for illustration purposes, and the location of the phase boundaries may depend on numerous system specific factors. The rate-dependent transition between capillary and viscous fingering is well documented [5] , [38] , [39] , and following Holtzman and Juanes [41] we depict the fracturing phase as rate independent. Our preliminary results suggest that the transition between frictional dynamics and fluidized front is largely ϕ independent (in our limited parameter space), whereas the boundary between corals (fluidized front) and viscous fingers is drawn slanted as the re-suspension process depends on the shear rate of the flow across the layer of settled material, and this shear rate increases with increasing ϕ as the free gap narrows. In conclusion, we find a remarkable variety of flow behaviour and displacement morphologies in frictional granular suspensions and poorly compacted granular media. Selected planes of the phase space have been mapped in detail, and transitions between various dynamic modes analysed in terms of the prevailing mechanisms and contending forces. As many geological fluid-particle flows happen in confinements, such as intrusion-fractures, lava-vents or the man-made hydro-fractures that are created for enhanced oil production, we expect natural realizations of our patterns to be found in contexts like these. Experimental setup The Hele-Shaw cell was constructed by bonding glass plates (350×350×10 mm 3 ) together using double sided tape along three sides, forming a 200×300×0.5 mm 3 channel. Another similar cell with plate thickness 19 mm was used for experiments requiring high stiffness to minimize the contribution to the total elasticity by bending of the plates. Loading of the granular dispersion and subsequent injection of air occurred through an inlet hole at one end of the channel, the opposite end being open. The granular material consisted of polydisperse glass beads of average diameter 100 μm. Most beads are spherical, but also present is a significant number of angular grains and smaller particles. The host fluid was a 50% water/glycerol solution. The added glycerol increases the viscosity of the host fluid such that the beads remain suspended during the injection, resulting in a fairly uniform distribution of the granular medium as it sediments on the lower glass plate. Air contained in a syringe was injected into the cell using a syringe pump (Aladdin, WPI) operated at a constant rate. The gas pressure was measured using a sensor (HCL0075D, Sensor Technics) connected to a DAQ system (NI cDAQ 9172, NI 9237, National Instruments). A camera (PL-B742U, Pixelink) placed underneath the cell captured time-lapse images. The cell was illuminated in brightfield mode using a white screen and two high-frequency linear fluorescent lights such that the granular material appears dark against a bright background. Data and image analyses were performed using standard commercial software. Theoretical model for the finger/bubble transition The fully mobilized frictional stress at the interface σ ( L ) takes the form [31] The mass density ρ is chosen as ρ =0.6( ρ g − ρ f ) where ρ g and ρ f are the mass densities of the glass that makes up the grains and the fluid, respectively, and 0.6 is the solid volume fraction of close-packed spheres. We use the following parameter values: ρ g =2400 kg m −3 , ρ f =1130 kg m −3 , μ =0.53, κ =0.8 and Δ z =0.5 mm. Mass conservation of the grains allows us to relate L and R c for a steadily advancing straight finger structure as L = ϕR c /(1− ϕ ). The capillary pressure along the front is P c ( R c )= γ / R c . We neglect the larger curvature associated with the transverse direction, as this is everywhere the same. The force balance on the interface at the finger tip is ΔP= γ / R c + σ ( R c ), and following ref. 31 we find the radius that minimizes this pressure, ∂/∂ R c ( γ / R c + σ ( R c ))=0, as where W is Lamberts W-function, that is, the inverse function of y = x e x . The half width of the resulting finger is found by equating the pressure at the tip and the straight sides, giving Having found the characteristic finger curvature as a function of ϕ , we consider the requirements for a transition to the bubble dynamics. We note that both the finger growth and bubble formation is a result of frictional stick-slip dynamics. We define the phase boundary between the two morphologies as the point where the expansion volume due to an individual slip event increases above , corresponding to a bubble of the same curvature as the finger tip. The transition point depends on (1) the frictional yield stress of the front, which increases with ϕ , and (2) the elastic response of the system, that is, the reservoir of air available for decompression, V air . For isothermal expansion of an ideal gas, we have that the product of pressure and volume is constant (Boyle's law), such that ( P 0 +Δ P )( V air –Δ V )= P 0 V air . As Δ P ≪ P 0 , we have Δ P /( P 0 +Δ P )≈Δ P / P 0 and therefore Δ P / P 0 ≈−Δ V / V air . We express the phase boundary as the minimum value of V air necessary to generate bubbles (equation (2)). Further, we use the ∂ P /∂ R c =0 condition to replace the exponential function in σ ( L ) (equation (5)) by noting that to express V air at the phase boundary as a function of ϕ and L (equation (3)). Transition from stick-slip to continuous dynamics When the injection rate is sufficiently large, the stick-slip dynamics of the bubbles will be replaced by continuous displacement. At the very least this requires that the particle packing in front of the fluid meniscus is fluidized before it reaches ϕ =1. However, although this is a necessary condition, the system still maintains its elastic response, which may allow the system to alternate between steady and stick-slip displacement. In other words, fluidization of the front before it reaches its close-packed value gives a lower bound on the critical injection rate needed for a transition to continuous motion. This condition may be formulated by the requirement that, at the front, the fluid forces exceed the friction caused by the weight of the particles. In mathematical terms, | ∇ P |> μρg , where ∇ P is now the fluid pressure gradient. By applying Darcy's law, ν =( k ( ξ )/( ξη ))| ∇ P |, where is the fluid velocity outside the bubble, ξ is the porosity, k ( ξ ) is the permeability of the packing and η the fluid viscosity, we may write We shall take the permeability to depend on ξ through the Kozeny–Carman relation k ( ξ )=( d 2 /180)( ξ 3 /(1− ξ ) 2 ), and use the close-packed porosity ξ =0.4. Further, the injection rate q is given by through , so, combining these results we get the critical injection rate This condition states that the packing is fluidized before it reaches a close-packed configuration. From direct observation it appears that the bubble sizes fluctuate around a value R =3 cm when Δ z =0.5 mm, and by using the parameter values η =0.01 Pa s, we find q c =0.05 ml min −1 . This value does not depend on ϕ or V air , although in practise the stability of the continuous motion will most likely depend on V air . How to cite this article: Sandnes, B. et al . Patterns and flow in frictional fluid dynamics. Nat. Commun. 2:288 doi: 10.1038/ncomms1289 (2011).